Stiff filamentous virus translocations through solid-state nanopores The ionic conductance through a nanometer-sized pore in a membrane changes when a biopolymer slides through it, making nanopores sensitive to single molecules in solution. Their possible use for sequencing has motivated numerous studies on how DNA, a semi-flexible polymer, translocates nanopores. Here we study voltage-driven dynamics of the stiff filamentous virus fd with experiments and simulations to investigate the basic physics of polymer translocations. We find that the electric field distribution aligns an approaching fd with the nanopore, promoting its capture, but it also pulls fd sideways against the membrane after failed translocation attempts until thermal fluctuations reorient the virus for translocation. fd is too stiff to translocate in folded configurations. It therefore translocates linearly, exhibiting a voltage-independent mobility and obeying first-passage-time statistics. Surprisingly, lengthwise Brownian motion only partially accounts for the translocation velocity fluctuations. We also observe a voltage-dependent contribution whose origin is only partially determined. A nanopore is a nanometer-scale hole in a thin insulating membrane that serves as a sensitive electronic detector. It senses when a single biopolymer threads it by registering a change in its ionic conductance [1] , [2] . The possibility of applying nanopores to the analysis of nucleic acids, in particular DNA sequencing, has generated interest [3] , and motivated fundamental studies of the physics of nanopore translocations [4] , [5] , [6] , [7] , [8] , [9] , [10] , [11] , [12] , [13] , [14] , [15] , [16] , [17] . The uses of solid-state nanopores have recently expanded to include detecting single proteins [18] , mapping structural features along RecA-bound DNA–protein complexes [19] and detecting spherical and icosahedral virus strains [20] , [21] , [22] . Such advances underline the importance of expanding our understanding of nanopore translocations beyond the case of DNA. A different approach is to study filamentous viruses, an interesting class of DNA–protein complexes with highly controllable physical and chemical properties. Filamentous viruses are also infectious agents that can be important targets for detection, as in the cases of the dangerous Filoviridae Marburg and Ebola [23] . The filamentous virus fd is a bacteriophage that infects Escherichia coli . Its contour length is L ≈880 nm [24] . A protein coat encases the single-stranded DNA genome, giving the virus a roughly circular cross-section with a diameter of 6.6 nm [24] , and a high negative linear charge density of −10 e nm −1 at pH 8.0 [25] , where e is the elementary charge. The monodispersity of fd makes it ideal for quantitative studies. In addition, fd can be chemically modified, and related virus strains are available with various lengths [26] , charge densities [27] and stiffnesses [28] . One can use fd to study the influence of stiffness on a filament’s capture by a nanopore and subsequent translocation. The persistence length of fd is P ≈2.8 μm [28] , which exceeds L by a factor of ∼ 3; fd therefore behaves like a stiff rod in solution rather than a random coil. By contrast, double-stranded DNA (dsDNA) has a persistence length of only ∼ 50 nm [29] . It is flexible enough to form hernias at the mouth of a voltage-biased nanopore, and translocate in a folded configuration [30] . Folded configurations are presumably suppressed when P exceeds some threshold. A polymer’s stiffness should also influence its translocation dynamics. According to the conventional theoretical picture, the electrokinetic driving force [10] , [12] , [13] and stochastic thermal forces [8] , [9] , [15] are balanced by the total viscous drag on the translocating polymer. The translocation is also retarded by electro-osmotic fluid flow through the nanopore [11] , [31] . The instantaneous drag includes a large contribution from the length of polymer moving towards the nanopore through solution [14] , [15] , [16] , [17] . Consequently, a DNA molecule that first threads the nanopore fully extended will experience more drag and translocate more slowly than if its initial configuration is a tight coil, close to the nanopore. The configuration of a dsDNA coil when it first threads the nanopore therefore determines its average translocation speed, υ [14] , [17] , and the distribution of initial configurations explains fluctuations in υ [15] . Fluctuations in υ are an impediment to using nanopores to size or sequence DNA. Here, we present experimental studies and simulations of the capture and translocation of fd in solid-state nanopores. To our knowledge, this is the first report of the translocation of stiff filaments of well-defined shape and size. We are able to distinguish fd ’s translocations and blunt collisions with the nanopore from the ionic current signal. The collisions, which are failed translocation attempts by a filament that is too stiff to enter the nanopore in a folded configuration, reveal a competition between electric and thermal forces in the capture process. Analysis of the translocations enables us to test theoretical models in an unexplored regime of polymer stiffness. Since fd is too stiff to coil, we expected its initial configurations and hence its mean translocation velocity to be more uniform than those of DNA. We expected the main source of velocity fluctuations to be the lengthwise Brownian motion of fd . We find that the dispersion in υ has two causes: translational Brownian motion of the stiff rod along its principal axis and a contribution that grows with voltage, whose possible origin we investigate with simulations and then discuss. Ionic current signatures of fd –nanopore interactions The basic principle of our experiments is illustrated in Fig. 1a . A nanopore in a 20-nm-thick silicon nitride membrane linked two reservoirs of buffered salt solution, across which a voltage, V , was applied, resulting in an ionic current through the nanopore, I . The filamentous shape and uniform charge of fd suit it well for interrogation by a voltage-biased nanopore, as illustrated in Fig. 1a . 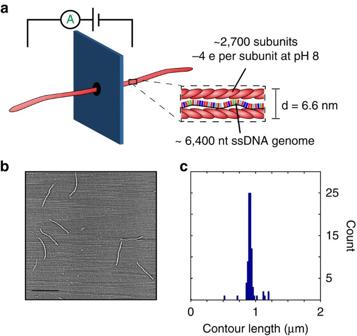Figure 1: Studies of filamentous viruses using nanopores. (a)fdvirus detection by a solid-state nanopore. The applied voltage draws a virus into the nanopore, where it blocks a measurable amount of ionic current. The detail sketches the single-stranded DNA (ssDNA) in its protein coat, which makesfdvirus 880 nm long and 6.6 nm wide, with a linear charge density of −10enm−1at pH 8.0. (b) AFM contact mode image offdvirus dried on a mica surface. Scale bar, 1 μm. (c) A histogram offdvirus lengths (N=87) as measured by atomic force microscopy. Figure 1b presents a typical atomic force micrograph of many fd viruses on a mica substrate. The distribution of L , obtained from multiple images and presented in Fig. 1c , shows a sharp peak at L ≈900 nm. After we introduced fd viruses into the negatively charged reservoir, they were electrophoretically drawn through the nanopore, causing transient changes in I . Figure 1: Studies of filamentous viruses using nanopores. ( a ) fd virus detection by a solid-state nanopore. The applied voltage draws a virus into the nanopore, where it blocks a measurable amount of ionic current. The detail sketches the single-stranded DNA (ssDNA) in its protein coat, which makes fd virus 880 nm long and 6.6 nm wide, with a linear charge density of −10 e nm −1 at pH 8.0. ( b ) AFM contact mode image of fd virus dried on a mica surface. Scale bar, 1 μm. ( c ) A histogram of fd virus lengths ( N =87) as measured by atomic force microscopy. 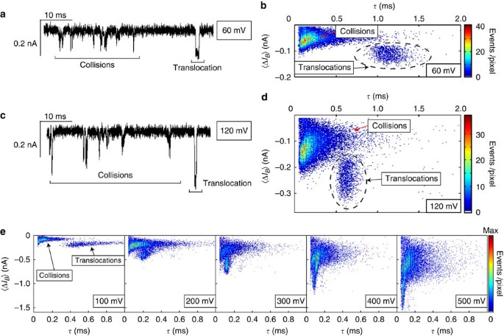Figure 2:Electrical signatures offdinteractions with a nanopore. Time traces ofI, recorded using a 26-nm-diameter nanopore, are shown for (a) 60 mV and (c) 120 mV. The buffer contained 200 mM KCl, 1 mM EDTA and 10 mM Tris–HCl (pH 8.0). Scatter plots show the events recorded at (b) 60 mV (3,565 events) and (d) 120 mV (4,704 events) from the same 26-nm-diameter nanopore. (e) Scatter plots of 〈ΔIB〉 versusτforVranging from 100 to 500 mV. The measurements used a 19-nm-diameter nanopore in 200 mM KCl. Full size image Figure 2a shows a typical time trace of I from a 26 nm-diameter nanopore, after fd virus was added to the negative reservoir. V was 60 mV and both reservoirs contained 200 mM KCl, pH 8.0 buffer. The open nanopore current was 6.2 nA. Blockages of I are distinguishable from the baseline; several minor blockages are followed by a sustained major blockage ≈0.12 nA in amplitude. Figure 2: Electrical signatures of fd interactions with a nanopore. Time traces of I , recorded using a 26-nm-diameter nanopore, are shown for ( a ) 60 mV and ( c ) 120 mV. The buffer contained 200 mM KCl, 1 mM EDTA and 10 mM Tris–HCl (pH 8.0). Scatter plots show the events recorded at ( b ) 60 mV (3,565 events) and ( d ) 120 mV (4,704 events) from the same 26-nm-diameter nanopore. ( e ) Scatter plots of 〈Δ I B 〉 versus τ for V ranging from 100 to 500 mV. The measurements used a 19-nm-diameter nanopore in 200 mM KCl. Full size image Figure 2b presents a scatter plot in which each blockage event is represented by a single point whose coordinates are given by the blockage duration, τ , and the mean current change during the blockage, 〈Δ I B 〉. (We obtained the instantaneous current change, Δ I B , by subtracting the mean of 4 ms of current on either side of a blockage event from I .) Two distinct populations of events can be seen. The first is centered around 〈Δ I B 〉≈−0.12 nA and τ ≈1.2 ms; it includes the major, sustained blockage in Fig. 2a , and ionic current signals similar to it. (More examples of major blockages are presented in Supplementary Fig. 1 ). The second population has smaller 〈Δ I B 〉 amplitudes and much shorter τ ; it includes the minor current blockages seen in Fig. 2a . (Our method for assigning each event to a particular population is described in the Methods.) Figure 2c shows a typical time trace obtained after raising the voltage to V =120 mV. Several minor blockages are again followed by a sustained major blockage. Figure 2d displays a scatter plot of the events observed with V =120 mV. Increasing V shifted the first population towards higher 〈Δ I B 〉 amplitude and lower τ ; doubling V approximately doubled 〈Δ I B 〉 and halved τ . The characteristic τ of the second population depended weakly on V , whereas its 〈Δ I B 〉 amplitude increased with V . Increasing V above 200 mV caused the two populations to overlap on a scatter plot, making them difficult to isolate. Scatter plots of events recorded with V ranging from 100 to 500 mV are presented in Fig. 2e . Events of each type tended to increase in frequency with V . Both populations shifted towards larger 〈Δ I B 〉 amplitudes with increasing ionic strength, roughly in proportion to the latter. (A comparison of events recorded at 200 mM KCl and 500 mM KCl is presented in Supplementary Fig. 2 ). Increasing the ionic strength to 300 mM or higher caused the two populations to significantly overlap. Such high salt concentrations also significantly increased the frequency of extremely long blockages that we attribute to fd clogging the nanopore. We deduce from multiple lines of evidence that the first population of events corresponds to translocations of the nanopore by fd . First, the regular time course of the events in that population was consistent with the insertion of a rod of uniform cross-section into the nanopore; those current traces were characterized by an abrupt, flat-bottomed blockage- a shape similar to the well-established signatures of linear DNA translocations [7] . Second, τ −1 and 〈Δ I B 〉 were proportional to V , as expected for electrophoretically driven translocations. Third, 〈Δ I B 〉 was approximately proportional to the salt concentration and its magnitude was in basic agreement with the theoretical model of Smeets et al. [4] , given the known diameter and linear charge density of fd (see Supplementary Note 1 ). Fourth, the range of τ was reasonable for fd translocations. We attribute the second population of events to side-on collisions of the virus with the nanopore. The minor blockage events in that population were characterized by lower 〈Δ I B 〉 and τ than translocations. We expect blunt collisions to block a smaller fraction of I than a virus that inserts fully into the nanopore. We frequently observed minor blockage events occurring in rapid succession before a translocation (see Supplementary Fig. 3 ). We interpret this pattern as a virus unsuccessfully attempting to translocate before thermal fluctuations present one of its ends to the nanopore and allow it to translocate. Such failed translocation attempts were observed in simulations, as we will discuss later. 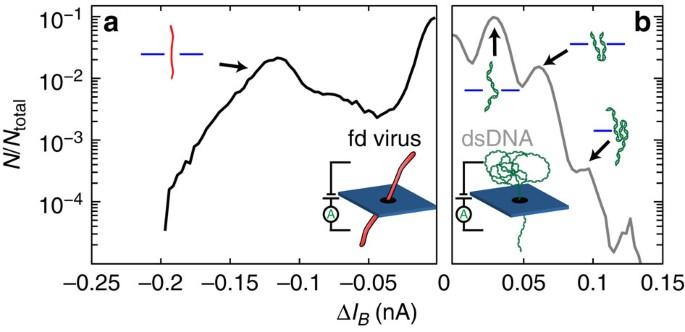Figure 3:Ionic current change caused byfdand dsDNA translocations. Histograms of the number of 4-μs-long samples of ΔIBper 3 pA bin (N), normalized by the total number of samples (Ntotal), forfd(panel (a), black, 280 translocations) and λ DNA (panel (b), grey, 1,434 translocations). The current recordings were performed on a 19-nm-diameter nanopore withV=100 mV in 100 mM KCl. The histograms represent currents recorded during translocation events and the 100 μs of baseline that preceded and followed each event. In 100 mM KCl,fdvirus translocations caused the current to decrease, whereas λ DNA caused it to increase. Positive (negative) values of ΔIBdue to baseline noise are omitted from thefd(λ DNA) histogram for clarity. Translocations through the nanopore Figure 3 compares histograms of 4-μs-long samples of Δ I B from translocations of the same 19-nm-wide nanopore by fd (black), and by L =16.5 μm, double-stranded λ DNA (grey), recorded in separate experiments. V was 100 mV. The electrolyte contained 100 mM KCl, a concentration at which fd and DNA translocations both produced observable ionic current changes. The DNA histogram reveals a series of approximately equally spaced blockage peaks at positive values of Δ I B , specifically 29±0.01, 61±0.04, 95±0.5 (a shoulder rather than a peak) and 125±0.7 pA. The fd histogram reveals a single major blockage peak at Δ I B ≈−115±0.2 pA. Figure 3: Ionic current change caused by fd and dsDNA translocations. Histograms of the number of 4-μs-long samples of Δ I B per 3 pA bin (N), normalized by the total number of samples ( N total ), for fd (panel ( a ), black, 280 translocations) and λ DNA (panel ( b ), grey, 1,434 translocations). The current recordings were performed on a 19-nm-diameter nanopore with V =100 mV in 100 mM KCl. The histograms represent currents recorded during translocation events and the 100 μs of baseline that preceded and followed each event. In 100 mM KCl, fd virus translocations caused the current to decrease, whereas λ DNA caused it to increase. Positive (negative) values of Δ I B due to baseline noise are omitted from the fd (λ DNA) histogram for clarity. 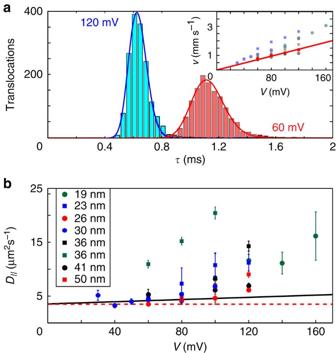Figure 4:fdtranslocation dynamics. (a) Distributions ofτforfdtranslocations of a 26-nm-diameter nanopore forV=120 mV (blue, 1,526 translocations) andV=60 mV (red, 1,223 translocations). The buffer contained 200 mM KCl. Solid lines are fits of equation (1). Inset: the dependence ofυonV. S.d. are comparable to the size of the symbols. The line is a linear fit to the data set represented in the histograms, fixed at the origin. (b) Dependence ofD||onV, from eight nanopores whose diameters are indicated. Error bars show s.d. found by bootstrap resampling of the data. The red dashed line showsD0,||, the lengthwise diffusivity offdin bulk solution. The black line plots the dependence ofD||onVobtained from simulations. Full size image Figure 4a shows the distributions of fd translocation times for V =60 and V =120 mV, from the 26-nm-wide nanopore considered in Fig. 2 . We quantified the translocation dynamics of fd with the one-dimensional Fokker–Planck equation, which yields the first-passage-time distribution [32] , [33] Figure 4: fd translocation dynamics. ( a ) Distributions of τ for fd translocations of a 26-nm-diameter nanopore for V =120 mV (blue, 1,526 translocations) and V =60 mV (red, 1,223 translocations). The buffer contained 200 mM KCl. Solid lines are fits of equation (1). Inset: the dependence of υ on V . S.d. are comparable to the size of the symbols. The line is a linear fit to the data set represented in the histograms, fixed at the origin. ( b ) Dependence of D || on V , from eight nanopores whose diameters are indicated. Error bars show s.d. found by bootstrap resampling of the data. The red dashed line shows D 0,|| , the lengthwise diffusivity of fd in bulk solution. The black line plots the dependence of D || on V obtained from simulations. Full size image We fit equation (1) to the measured τ distributions using υ and D || as fitting parameters. F ( τ ) is the probability density for a one-dimensional walker with drift velocity υ and dispersivity D || to travel a distance L for the first time in an interval τ . Good fits of equation (1) to the data were obtained for all V . The dependence of υ on V , plotted in the inset of Fig. 4a , is well fit by a line passing through the origin. The slope of the line obtains the mobility of fd in the nanopore, μ fd ,pore =1.2±0.1 cm V −1 s −1 . The mean mobility in the eight nanopores tested at 200 mM KCl was 〈 μ fd ,pore 〉=1.4±0.4 cm V −1 s −1 . The widths of the τ distributions arise from fluctuations of the translocation velocity, which we quantify with the fit parameter D || . The voltage-dependence of D || is plotted in Fig. 4b for eight nanopores. For comparison, the figure also shows the diffusion coefficient of fd for lengthwise motion, D 0,|| =3.5 μm 2 s −1 (see Methods). The measured values of D || were typically close to D 0,|| for V ≤60 mV. D || began increasing with V beyond about 60 mV. By V =120 mV, D || exceeded D 0,|| by a factor of 2–4. The rise in D || was accompanied by a widening spread in values measured on different nanopores. We did not find a clear relationship between D || and the size of the nanopore. In all nine nanopores with diameters under 15 nm that we tested with fd , the virus repeatedly stuck inside the nanopore, making it difficult to observe a significant number of translocations. We also found no difference in the behaviour of D || , within experimental error, between fd ’s translocations and those of an even stiffer mutant, fd -Y21M (see Supplementary Fig. 4 ; Supplementary Note 2 ). We performed simulations to investigate possible sources of translocation velocity fluctuations, including the incident angle of the virus on first entering the nanopore, the influence of the electrophoretic forces acting on the virus outside the nanopore and the bending of the finitely deformable virus. Our simulations used coarse-grained Langevin Dynamics [41] . We modelled fd as a generic linear polymer composed of 133 beads of diameter σ , giving the correct aspect ratio. We imposed a persistence length of P =423 σ , such that P =3.2 L , as with fd . We solved the electric potential via a finite difference approach for the nanopore geometry to account for the electric forces inside and outside the nanopore. We simulated different driving forces by multiplying the potential distribution by a constant scaling factor, λ . We matched simulation and experimental forces by matching the balance between drift and translational diffusion, given by the Péclet number for lengthwise motion, . Pé is a convenient and meaningful measure of the driving force in simulations [42] . In our simulations, D 0,|| = D 0 (the diffusivity and the lengthwise diffusivity are equal), because hydrodynamic interactions are ignored. See Methods for further details. 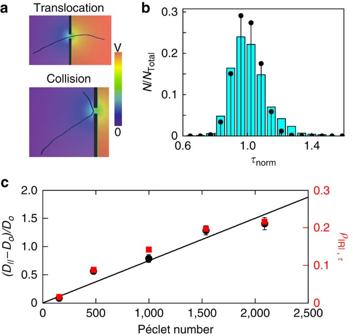Figure 5:Simulations offdtranslocations. (a) Examples of a translocation (top of panel) and a collision (bottom of panel). The background colour maps the electric potential distribution. (b) Distributions ofτ, normalized byL/υ. Black stems represent 3,751 simulated translocations withPé≈480. Cyan bars represent 1,526 experimentalfdtranslocations of a 26-nm-diameter nanopore withV=120 mV, for whichPé≈357. (c) Dependence of (D||−D0)/D0(black) andρ|R|,τ(red) on Pé. Error bars show s.d. obtained by bootstrap resampling of the data. The black line is a linear fit, fixed at the origin, to (D||−D0)/D0as a function ofPé. Figure 5a presents sample images from the simulations. The upper image shows a simulated polymer translocating the nanopore; the lower one shows a simulated polymer colliding with the nanopore side-on. Its high stiffness prevented it from forming a hernia and translocating in a folded configuration. The background colours indicate the potential distribution. It has a large gradient outside the nanopore, which draws in the simulated polymer. The force gradients also exert a torque on the simulated polymer that tends to align it with the nanopore. Figure 5: Simulations of fd translocations. ( a ) Examples of a translocation (top of panel) and a collision (bottom of panel). The background colour maps the electric potential distribution. ( b ) Distributions of τ , normalized by L / υ . Black stems represent 3,751 simulated translocations with Pé ≈480. Cyan bars represent 1,526 experimental fd translocations of a 26-nm-diameter nanopore with V =120 mV, for which Pé ≈357. ( c ) Dependence of ( D || − D 0 )/ D 0 (black) and ρ | R |,τ (red) on Pé. Error bars show s.d. obtained by bootstrap resampling of the data. The black line is a linear fit, fixed at the origin, to ( D || − D 0 )/ D 0 as a function of Pé . Full size image Equation (1) was fit to distributions of τ obtained from simulations. The resulting υ was proportional to the simulated force and Pé , to a very good approximation. Figure 5b compares distributions of τ from simulations and an experiment with similar values of Pé . τ was normalized by the corresponding L / υ in each distribution. The simulation distribution is sharper than the experimental one, but similar in other respects. Our fits of equation (1) to the simulation distributions also revealed that D || increased with the driving field. Figure 5c plots the fractional enhancement of D || above D 0 , ( D || − D 0 )/ D 0 , as a function of Pé . The increase in ( D || − D 0 )/ D 0 with Pé is well fit by a line passing through the origin. We make a quantitative comparison between simulations and experiments in Fig. 4b . We fit a line to the simulation results in Fig. 5c , set D 0,|| (= D 0 in simulations) to 3.5 μm 2 s −1 and converted Pé to V using Pé =( L 〈 μ fd ,pore 〉/ D 0,|| ) V . We found that V =(48.7±9.0 mV) × λ , (see Methods). Figure 4b plots the resulting relationship between D || and V (black line), extrapolated from simulations. Compared with experiments, simulations showed a much slower rise in D || with V . Collisions with the nanopore Our ability to separate fd ’s translocations through the nanopore from its collisions against it enables us to investigate the capture process. We are particularly interested in the efficiency with which the nanopore captures a virus by its end, which is not much smaller than the nanopore itself, relative to failed translocation attempts. It is difficult to count translocation attempts, however, because the result depends on how one distinguishes or groups collision events that occur in rapid succession. Furthermore, we do not know whether two translocation attempts were by the same virus. To avoid these difficulties, we quantify collisions and translocations by their event charge deficit (ECD). ECD is the change in ionic current caused by an event, integrated over the duration of that event [6] . The total ECD of all collisions, ∑ ECD Col , is a useful measure of translocation attempts, and can be compared with the total ECD of all translocations, ∑ ECD Trans . 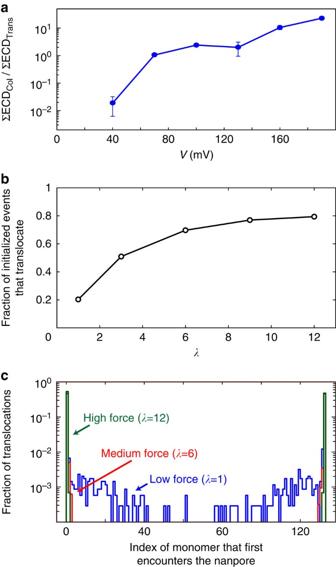Figure 6: Translocation attempts. (a) The ratio of the total ECD from collisions to the total ECD from translocations plotted as a function ofV, from a representative experiment on a 28-nm-diameter nanopore in 200 mM KCl. Errors were calculated by bootstrap resampling. (b) The fraction of initialized simulations that ended with a successful translocation as a function ofλ. (c) Histograms of the index of the first monomer to encounter the nanopore for successful translocations withλ=1 (blue),λ=6 (red) andλ=12 (green). The simulated polymer was 133 monomers long. Figure 6a plots the dependence of the ratio ∑ ECD Col /∑ ECD Trans on V . The ratio increased with V . For the lowest applied voltages, ∑ ECD Col was significantly smaller than ∑ ECD Trans . At the high end of the applied voltage range, the situation was reversed, and collisions were the dominant source of ECD. Figure 6: Translocation attempts. ( a ) The ratio of the total ECD from collisions to the total ECD from translocations plotted as a function of V , from a representative experiment on a 28-nm-diameter nanopore in 200 mM KCl. Errors were calculated by bootstrap resampling. ( b ) The fraction of initialized simulations that ended with a successful translocation as a function of λ . ( c ) Histograms of the index of the first monomer to encounter the nanopore for successful translocations with λ =1 (blue), λ =6 (red) and λ =12 (green). The simulated polymer was 133 monomers long. Full size image We also investigated the capture efficiency with simulations. Figure 6b plots the fraction of simulated polymers that translocated successfully within the allotted ≈8-ms window against λ , the simulation force-scaling parameter. The fraction of captures increased with λ . Figure 6c shows histograms of the index of the first monomer of the simulated polymer to encounter the nanopore for each translocation, for three different values of λ . A monomer was judged to have encountered the nanopore if it came within 2.5 σ of the center of the nanopore. For high and medium λ , successful translocations only occurred if the simulated polymer approached the nanopore end-on (see also Supplementary Fig. 5 ; Supplementary Fig. 6 ). At low λ , on the other hand, the simulated polymer frequently approached the nanopore side-on, had a monomer far from its ends collide with the nanopore, but was still able to reorient and translocate within the time window. Magnitude of the ionic current changes The peaks in the experimental Δ I B histograms ( Fig. 3 ) report the relative frequencies of folded configurations of the translocating filaments. The high intensity at Δ I B =0 pA in both histograms corresponds to current through the open nanopore. The first peak in the DNA histogram is caused by the presence of a single segment of DNA inside the nanopore. The second, third and fourth peaks correspond to DNA folded once, twice and three times, respectively, because each additional strand occupying the nanopore causes an incremental change in I . Similarly, the peak in the fd histogram at Δ I B ≈−115 pA is due to linear translocations. The absence of an additional peak at Δ I B ≈−230 pA indicates that fd never translocated in a folded configuration. The sign and magnitude of Δ I B are determined by two competing effects: an enhancement of the current carried by counterions along the charged filament, and a reduction in the current carried by bulk ions proportional to the conductivity of the electrolyte and the cross-sectional area of the filament [4] . Both effects are proportional to V . Translocations are expected to cause current blockages at high ionic strength, and current enhancements at low ionic strength, with a crossover at ≈370 mM KCl for dsDNA [4] . Accordingly, we observed a current enhancement of Δ I B ≈29 pA for dsDNA at 100 mM KCl. In the case of fd , the viral cross-section exceeds that of dsDNA by a factor of ∼ 9, strongly favouring current blockages, despite its high linear charge density, which is ∼ 1.7 times that of dsDNA. These properties lead to the rough estimate of a crossover from current blockages to enhancements at 70 mM KCl for fd , in agreement with our observation of current blockage at 100 mM KCl. The theoretical model of Smeets et al. [4] predicts Δ I B ≈−77 pA for dsDNA and Δ I B ≈−170 pA for fd (see Supplementary Note 1 ), whose signs and magnitudes are in reasonable agreement with the measured values for dsDNA (≈29 pA) and fd (≈−115 pA). The discrepancies between theory and experiment are likely traceable to two phenomenological fitting parameters on which that model relies: a Manning condensation parameter that accounts for the reduced mobility of tightly bound counterions, and an effective pore length that accounts for the geometry of the nanopore. Further studies of fd could lead to a better understanding of these important but poorly understood effects. The translocation velocity A linear dependence of υ on V , observed in Fig. 4 , is expected for fd translocations. The applied voltage drives the virus with an electrophoretic force and with electro-osmotic flow generated within the charged walls of the nanopore, both of which are linear in V . Those driving forces are balanced by Stokes drag, which is linear in υ [10] , [11] . The mobility of fd is difficult to compute accurately because it depends on the detailed geometry and charge distribution of the nanopore and of the virus. If we instead compare the mobility of fd to that of λ DNA translocating under similar conditions ( μ DNA,pore ≈11 cm V −1 s −1 ), we find that the latter is a factor of 7 higher. We can account for that difference by considering the factors that are theoretically understood to affect the translocation speed. First, we note that the mobility of dsDNA in bulk electrolyte is almost three times higher than for fd ( μ DNA =3.75 × 10 −4 (ref. 34 ) versus μ fd =1.3 × 10 −4 cm 2 V −1 s −1 (ref. 35 ), respectively). Second, since silicon nitride nanopores are negatively charged at pH 8.0, translocations of DNA and fd will both be slowed by the same electro-osmotic slip speed, which will amplify the relative difference in their mobilities. Third, the stiff fd virus has a higher viscous drag coefficient than λ DNA, and that contributes to the slower translocation speed of fd . Viscous drag is felt by whatever part of the polymer is being pulled toward the nanopore through the fluid. That length is different for fd and λ DNA. For λ DNA, the translocation process is typically fast compared with the relaxation time of the coil. The translocating polymer can therefore be thought of as a dormant portion that experiences no drag, and a moving segment that does [36] . The dormant portion includes the relaxed coil awaiting translocation near the nanopore, and the segments of DNA accumulating on the opposite side after translocating the nanopore. The moving segment is the part under tension as it is drawn towards the nanopore [14] , [15] . The length of the moving segment is approximately the radius of gyration of the polymer coil, ≈730 nm for λ DNA [37] . (This approximation likely overestimates the characteristic length because it ignores the effect of the trailing end [17] ). The diameter of the moving segment is that of the DNA double helix, 2.2 nm, because that segment is under tension. For fd , which is much stiffer, the entire contour length is the moving segment and there is no dormant portion on either side of the nanopore. The length and diameter of fd result in a drag coefficient that is about 1.7 times higher than that of the moving segment of λ DNA, as calculated for slender rods. In summary, a comparison with DNA shows that the mobility of fd in nanopores is consistent with its distinct physico-chemical properties. The mobility varied from nanopore to nanopore with a s.d. of 33%, as shown in the inset of Fig. 4a . We speculate that differences in the surface charge of the nanopores partly explain this variation. Differences in the shape of the electric field lines inside the nanopores due to surface roughness or variations in how the nanopore was drilled or cleaned could also explain the spread in mobilities. Velocity fluctuations Equation (1) describes the distributions of fd translocation times well (for example, Fig. 4a ). That equation presumes a Gaussian distribution of velocity fluctuations, but it makes no assumptions about their physical origin. The lengthwise Brownian motion of fd is a fundamental source of velocity fluctuations that undoubtedly contributes to D || . Nevertheless, it is possible for D || to be lower than D 0,|| ; it was recently reported that small, spherical proteins translocating through nanopores exhibited a diffusivity that was voltage-independent and 50 times lower than the bulk diffusion coefficient, a result attributed to confinement and interactions between the protein and the nanopore [39] . D || can also exceed D 0,|| , as in Taylor–Aris dispersion [38] . We have considered these and other possible sources of dispersion, which are discussed below. The lengthwise Brownian motion of fd set a lower bound to the velocity fluctuations. Figure 4b shows that D || did not fall below D 0 , within error. D || was typically close to D 0,|| for V ≤60 mV. For V ≥100 mV, D || increased beyond D 0,|| with V . This indicates that there must be a source of velocity fluctuations that is distinct from lengthwise Brownian motion and that depends on the driving force in some fashion. We used simulations to investigate different mechanisms that could account for this extra contribution to D || . Specifically, we examined the correlations between τ and the simulated polymer’s angular orientation at the onset of translocation, its lateral position inside the nanopore and the flexing of the polymer at the onset of translocation. We found no significant correlation between τ and the orientation of the simulated polymer, or its lateral position in the nanopore. We found a positive correlation between τ and the end-to-end distance of the simulated polymer at the onset of translocation, | R | (see Supplementary Fig. 7 ). We quantified that correlation by the Pearson product-moment correlation coefficient, ρ | R |,τ , and plotted its dependence on Pé in Fig. 5c . ρ | R |,τ increased approximately linearly with Pé . The dependence of ρ | R |,τ on Pé was almost identical to that of ( D || − D 0 )/ D 0 . The large but finite persistence length allowed the simulated polymer to adopt a variety of bending configurations. A bent configuration at the start of a translocation brings the monomers closer to the nanopore, on average, than an extended configuration. Consequently, the monomers of bent polymers initiate translocations from regions of relatively high force and their short distance to the nanopore results in low fluid drag during translocation. Those two mechanisms explain the decrease in τ we observed with increasing amounts of initial bending, quantified by ρ | R |,τ in simulations. Velocity fluctuations increase with Pé because stronger driving forces give diffusion less opportunity to wash out the initial condition of the polymer. The strongest force gave translocation times ( τ ≈1,000) similar to the simulated polymer’s longest relaxation time (637 in simulation units, see Supplementary Fig. 8 ). When we simulated a polymer with the same high persistence length as the fd -Y21M strain, we found its D || was lower than that of fd for a given Pé , as expected. The differences in D || were small, however, because fd is very stiff, so its bending configurations are already significantly limited (see Supplementary Fig. 4 ; Supplementary Note 2 ). We conclude that the voltage-dependent dispersion in τ seen in simulations was caused by variations in the initial bending configuration of the simulated polymer. When compared quantitatively with experiments in Fig. 4b , however, simulations showed a much slower rise in D || with V . This indicates that the spread in the viruses’ initial bending configurations explains only part of the rise in D || with V . The additional velocity fluctuations of fd at high V must occur by a mechanism not modelled in our simulations. One possibility is that the pulling force depends on the lateral position of the virus inside the nanopore, which drives a mechanism similar to Taylor dispersion [38] . Since fd diffuses laterally inside a nanopore, each virus trajectory would sample the pulling forces differently, leading to additional velocity fluctuations. In a typical translocation, fd diffuses laterally by 60 nm on average, which is about twice the diameter of the nanopore if we assume D 0, ⊥ =2.1 μm 2 s −1 and τ =1 ms. The velocity fluctuations should grow with V because fast translocations limit the virus’s chance to sample the force landscape. It was recently proposed by Lu et al. [12] that the net electrokinetic force (on DNA) does in fact depend on the lateral position of the polymer. That detailed electrokinetic force model was not included in our simulations. Another possibility is the friction between the virus and the nanopore wall. If a virus enters the nanopore obliquely, the electric fields will push the virus against the side of the nanopore and friction will rise. This could create a strong dependence of the translocation time on the angle, with oblique angles expected to generate more friction than if the virus is parallel to the axis of the nanopore. Lower voltages would give more time for rotational diffusion to wash out the effect of the initial angle, leading to a rise in D || with V . Our simulations did not include chemical interactions that can generate strong friction. They showed no influence of the angle on the translocation dynamics. Capture of fd by the nanopore Our experimental and simulation results paint a coherent picture of the capture of fd by the nanopore. We interpret those results as follows. Figure 6a shows a rapid growth in collisions relative to translocations as the voltage was raised. Viruses that became trapped sideways by the electric fields were in a metastable state, and required thermal activation to reorient and translocate. Figure 6a indicates that viruses were drawn ever tighter to the nanopore by the increasing electric fields. This interpretation is also consistent with our observation that collisions increased in frequency with increasing salt concentration (see Supplementary Fig. 2 ). A higher salt concentration reduced the repulsion between the negatively charged virus and the silicon nitride surface, leading to more collisions. The simulation results in Fig. 6b show an increasing frequency of successful translocation attempts with voltage. This result reflects the tendency of the electric field gradients to orient an approaching virus towards the nanopore. Experimentally, the rate at which the nanopore captured fd also increased with V , partly for the same reason, we expect. Finally, Fig. 6c shows that successful translocations grow increasingly infrequent with applied force unless the approaching polymer first makes contact with the nanopore near or at its very end. This result illustrates the dual role played by the electric fields, aligning the approaching molecule on one hand, and trapping a molecule after a failed translocation attempt on the other. We note that typical experimental voltages correspond to low values of λ ( V =(48.7±9.0 mV) × λ , see Methods). In this regime, the electric forces are less likely to attract the virus to the nanopore end-on, but thermal fluctuations enable it to reorient and translocate after failed attempts. There is an important qualitative difference between the minor current blockages caused by fd collisions and the minor current blockages recently observed with DNA, which were also interpreted as collisions with the nanopore [43] , [44] , [45] , [46] . The DNA collisions reportedly led quickly and reliably to a translocation, whereas fd collisions were not always followed by a translocation. We believe this is because fd is orders of magnitude stiffer than dsDNA and thus forbidden from being captured in a folded configuration, unlike DNA. We studied the filamentous virus fd to understand the physics of stiff polymer translocations. Our experiments and simulations reveal an interesting interplay between thermal fluctuations and the electric fields outside the nanopore, which determines the capture of fd viruses. The electrophoretic forces tend to align a virus towards the nanopore, facilitating the capture of an approaching virus. If the virus fails to insert its end into the nanopore, however, the same electric fields tend to trap the virus sideways against the nanopore membrane. The electric fields pull the virus harder against the membrane as the applied voltage grows, and it becomes increasingly rare that thermal fluctuations reorient the virus in a way that allows it to translocate. fd was too stiff to enter the nanopore in a folded configuration. The translocation times of fd obey first-passage-time statistics, which are useful for quantifying the mean drift velocity and the dispersivity. The velocity of fd is linear in the applied voltage, and consistent with its physical and electrical properties when compared with DNA within the current theoretical picture. The lengthwise Brownian motion of fd is a fundamental source of velocity fluctuations that sets the floor on the value of fd ’s dispersivity. We discovered an additional, voltage-dependent source of velocity fluctuations that grew increasingly important at high voltages. Langevin dynamics simulations show a correlation between the initial bending configuration and the translocation speed, which grows with voltage. The distribution of initial configurations therefore gives rise to velocity fluctuations, but only a small fraction of what was measured experimentally. There remains an additional source of velocity fluctuations whose origin is not yet properly understood. Finally, we speculate that the label-free detection of fd might have practical applications, as fd virus is a marker of sewage contamination in ground water [47] , and of E. coli contamination of the food supply [48] . Experimental procedures Nanopores were pierced through 20-nm-thick membranes made of low-stress LPCVD silicon nitride using a JEOL 2010F or a JEOL 2100F high-resolution transmission electron microscope. The detailed fabrication procedure can be found in ref. 49 . The transmission electron microscope was also used to measure the diameter of the nanopore. We tested nanopores with diameters ranging from 12 to 50 nm. Each nanopore was cleaned with Nano-Strip (Cyantek) for 2 h at 75 °C before use. The nanopore was then mounted in a custom-made fluidic cell. fd virus was grown and purified according to standard biological procedures [50] , using Xl1-Blue as the host E. coli strain. Virus samples were prepared in high concentrations in 100 mM NaCl, 20 mM Tris, pH 8.0 buffer, and then diluted to a 0.02 mg ml −1 (≈1 nM) virus concentration in the desired buffer solution. The overlap concentration of fd virus is 0.11 mg ml −1 (≈5 nM) [51] , so we assume no interaction between fd particles. We prepared samples of similar concentration for the λ DNA measurements. These samples were also far below the overlap concentration for a worm-like chain with the same length as λ DNA (48.5 kbp or 16.5 μm) [51] . Buffer solutions at pH 8.0 were prepared using de-ionized water (Millipore), with 10 mM Tris, 1 mM EDTA and a variable KCl concentration. The buffer solutions were vortexed for 30 s to disperse the viruses before adding them to the negative chamber of the fluidic cell. Ag-AgCl electrodes were immersed in both chambers of the fluidic cell and connected to an Axon Axopatch 200B current amplifier, which maintained a constant potential difference while monitoring I . The signal was conditioned by an 8-pole Bessel filter with a cutoff frequency of 10 or 50 kHz, and then digitized using a 250-kHz sampling rate. Samples of fd on mica were imaged by atomic force microscopy (AFM) using a Dimension 3100 microscope (Digital Instruments) operating in contact mode. MATLAB was used to threshold the AFM images, measure the contour lengths of the fd filaments and correct for tip-broadening. Estimation of D 0,|| for fd virus We estimated D 0,|| from the diffusion coefficient of fd in aqueous buffer at 25 °C, D 0 =2.58 μm 2 s −1 (ref. 52 ), the relationship between the parallel and perpendicular components of the diffusion coefficient, D 0,|| and D 0, ⊥ , respectively, for a rigid rod of finite length and width [40] , and the relationship D 0 =(2 D 0, ⊥ + D 0,|| )/3. Event extraction and classifications The analysis of ionic current recordings was performed in two stages using custom MATLAB programs. In the first stage, a program identified the approximate locations of all significant blockage events in the current recordings. In the second stage, a different program determined the precise times of the start and end of each event, and then performed an analysis on the current blockage amplitudes over the course of each event. The event-identification program stepped a 255-data-point window through the time-ordered current samples point by point, comparing the leading 5 data points (20 μs) to the trailing 250 data points (1 ms), which represent the baseline. When the mean value of the leading section fell below the mean value of the baseline by some threshold amount, the program classified that current fluctuation as an event. The threshold parameter was adjusted depending on the noise characteristics of the current recording. A typical threshold value was 10 times the r.m.s. noise level. A lower threshold was occasionally used when it appeared that translocations were being missed because they were below the threshold, based on a visual inspection of the data. The end of an event was by the mean value of the test section approaching the original baseline level to within 10% of the r.m.s. noise level. In this manner, the event-identification program quickly scanned the raw data and determined the tentative start and end times of events. We developed a separate, more computationally intensive program to precisely define the start and end times of events, and to analyse characteristics of those events. That program focused on the events identified in the first stage, plus the 200 data points (0.8 ms) on either side of each event. The program first smoothed the current using a moving average of five data points, then computed the second derivative of the smoothed current numerically. The precise start and end of an event were defined as the minima occurring within 180 μs of the tentative start and end times, respectively. (According to this definition, the start of an event corresponds to when the current first leaves the baseline, and the end when it first returns to the baseline). This method determined the start and end times of fd translocations accurately and reliably even in the presence of frequent collision signals, and without employing an arbitrary current threshold. These features were important for obtaining robust measurements of D || across different experimental conditions. Each event was classified as either a collision or a translocation based on its ECD value [6] . ECD is the integrated current change from the local baseline over the duration of the event. 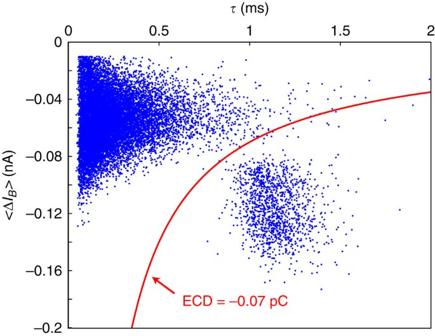Figure 7: Separating translocations from collisions. Scatter plot of 〈ΔIB〉 versusτfor 3,565 events recorded using a 26-nm-diameter nanopore, withV=60 mV, in 200 mM KCl, pH 8.0 buffer. The red line indicates the constant ECD=−0.07 pC value used as the boundary between translocation events and collision events. Figure 7 shows a scatter plot of events in terms of 〈Δ I B 〉 and τ from the same V =60 mV recording presented in Fig. 2 . A line indicating ECD=−0.07 pC is also plotted in Fig. 7 . Events below the line (|ECD|>0.07 pC) belong to the translocation population, and those above it (|ECD|<0.07 pC) belong to the collision population. Since collisions tend to be shorter than translocations, it is possible they were attenuated owing to the bandwidth limitations of our electrometer. This could decrease the apparent |ECD| of collisions. For some experiments, a filter was applied to remove outliers characterized by low 〈Δ I B 〉 and high r.m.s. noise levels from the translocation population; we interpret long-lived events with low 〈Δ I B 〉, which yield a high |ECD|, as the products of unusually long collisions, rather than translocations. An additional cutoff was necessary for some higher voltages ( V ≥160 mV). At these voltages, collisions often appeared in quick succession. The current values just before and after (within 0.1 ms) these collisions, or the local baseline, were often lower than the open pore current. Translocations were more likely to have local baselines equal to the open pore current. If an event had a local baseline that was lower than the open pore current, within noise, the event was classified as a collision. Figure 7: Separating translocations from collisions. Scatter plot of 〈Δ I B 〉 versus τ for 3,565 events recorded using a 26-nm-diameter nanopore, with V =60 mV, in 200 mM KCl, pH 8.0 buffer. The red line indicates the constant ECD=−0.07 pC value used as the boundary between translocation events and collision events. Full size image We note here that we have excluded outliers in event duration for Fig. 3 ( τ ≥1 ms) to discount any stuck viruses. In addition, we low-pass filtered the current in this data set with an additional 20-kHz-low-pass software filter to remove digitization noise, so that we could employ a finer bin size. Since the data were originally collected with a 10-kHz-low-pass hardware Bessel filter, this software filter did not affect the appearance of the folding peaks apart from the removal of digitization noise. We also note that all collisions with |ECD|’s >6 s.d. away from the mean |ECD| were excluded from Fig. 6a to avoid including clogs. The same was done with translocations in Fig. 6a . Langevin dynamics simulations of fd translocations We used a standard coarse-grained approach to model the fd virus as a polymer consisting of 133 monomers of size σ [41] . We bound adjacent monomers together by the finitely extensible nonlinear elastic potential: where we set the spring constant k to 30 ∈ / σ 2 (with ∈ being the characteristic energy) and the maximum extension r 0 to 1.5 σ as in the model of Kremer and Grest [53] . A shifted and truncated Lennard-Jones potential often called the WCA potential [54] gave the excluded volume interactions between monomers: where the cutoff distance r c was set to 2 1/6 σ . We implemented the persistence length by a bending potential given by where θ is the angle formed by three consecutive monomers, k is the spring constant and θ 0 is equilibrium angle. To model fd virus, we set θ 0 to 180° and k =423, yielding a persistence length of 423 σ and giving the correct ratio of persistence length to contour length. We used a continuous surface of thickness 3 σ for the membrane. The diameter of the cylindrical nanopore was d pore =5 σ , corresponding to a typical experiment, where d pore ≈30 nm and l pore ≈20 nm. The details of the potential resulting from applying a voltage drop of Δ V across this geometry were solved via a finite difference approach. For computational efficiency, the simulations did not explicitly include solvent. Instead, we used a Langevin Dynamics approach in which the effects of the solvent are included implicitly by including both a damping term and a random force term directly in the equation of motion. The final equation of motion is then given by where m is the monomer mass, F ext is the external force, U ( r ) is the sum of the conservative potentials ( U FENE ( r ), U WCA ( r ) and U bend ( θ )), ζ is the friction coefficient and ξ ( t ) is the random force term. ξ( t ) satisfies the following criteria: in accordance with the fluctuation-dissipation theorem. F ext was adjusted using a scaling parameter, λ , to change the applied force on the simulated polymer. Simulation forces were matched to experimental conditions by ensuring the balance between drift and diffusion was the same in simulations as in experiments. This balance was calculated via a translocation Péclet number defined as Pé = L υ/ D =(( L 〈 μ fd ,pore 〉)/( D 0,|| )) V . We measured the experimental mobility of fd virus translocations to be 〈 μ fd ,pore 〉=14.0±3.8 mm V −1 s −1 . Using the known length of fd virus and its diffusion coefficient, D 0,|| =3.5 μm 2 s −1 , we obtained Pé exp =(3.52±0.95) × 10 3 V , where V is the applied voltage in volts. For V =100 mV, Pé exp =352±95. We applied a similar method to determine the simulation Péclet number. We measured the simulation mobility to be 〈 μ sim 〉=(9.7±0.28) × 10 −3 a.u. The simulation length, L , is N =133, while the diffusion coefficient D sim =1/ N . We obtained Pé sim =(172±05) λ . Matching Pé exp and Pé sim , we find that V =(48.7±9.0 mV) × λ . Simulations were performed using the ESPResSo package [55] on the SHARCNET computer system ( http://www.sharcnet.ca ) using visual molecular dynamics [56] for visualization. How to cite this article: McMullen, A. et al. Stiff filamentous virus translocations through solid-state nanopores. Nat. Commun. 5:4171 doi: 10.1038/ncomms5171 (2014).